Dysregulation of hydrogen sulphide metabolism impairs oviductal transport of embryos Embryo retention in the fallopian tube is thought to lead to ectopic pregnancy, which is a significant cause of morbidity. Hydrogen sulphide (H 2 S) is a gaseotransmitter produced mainly by cystathionine-γ-lyase and cystathionine-β-synthase. Here we show that cystathionine-γ-lyase and cystathionine -β-synthase are ubiquitously distributed in human fallopian tube epithelium and that H 2 S signalling relaxes the spontaneous contraction of the human oviduct. Furthermore, an aberration in H 2 S signalling, either silenced or enhanced activity induced by pharmacologic or genetic methods, causes embryo retention and developmental delay in the mouse oviduct, which is partly reversed by administration of either GYY4137, a slow-releasing H 2 S donor, or NaHS. Our findings reveal a new regulatory mechanism for oviductal embryo transport. Hydrogen sulphde (H 2 S) is considered the third member of the gaseotransmitter family, along with nitric oxide (NO) and carbon monoxide (CO) [1] . Physiologically, H 2 S is generated from L -cysteine in reactions catalysed by three enzymes, including cystathionine-γ-lyase(CSE), cystathionine-β-synthase(CBS) [1] , [2] and 3-mercap-topyruvatesulphurtransferase (3MST) [3] . Both CBS and CSE are localized to the cytoplasm, whereas 3MST is localized predominantly to the mitochondria. CSE is primarily responsible for most of the H 2 S production in the vasculature [4] , [5] , whereas CBS may be primarily responsible for H 2 S formation in the brain. H 2 S produced by 3MST regulates mitochondrial reactive oxygen species (ROS) production [3] . Intriguingly, the expression of H 2 S-generating enzymes and the endogenous production of H 2 S have recently been identified in male and female reproductive systems in several mammalian species [6] , [7] , [8] , [9] , [10] , [11] . In the male reproductive duct, endogenously produced H 2 S mediates erectile function [7] , [12] , [13] , [14] , spermatogonial proliferation [6] and vas deferens smooth-muscle relaxation. CBS and CSE have also been detected in the female reproductive tract and gestational tissues, including the uterus and vaginal, placental and fetal membrane tissues [9] , [10] , [15] . In our present study, we demonstrated that CBS and CSE are ubiquitously distributed in human fallopian tube epithelium and that H 2 S signalling mediates the spontaneous contraction of human oviduct and oviductal embryo transport. We also found that aberrant H 2 S signalling impaired oviductal transport of embryos and preimplantation embryo development, which was restored by administration of H 2 S. Intriguingly, H 2 S signalling is upregulated in an ectopic pregnancy. In addition to uncovering a new regulatory mechanism, this study could be clinically relevant to ectopic pregnancy. A H 2 S generation pathway exists in human fallopian tubes First, we performed immunoblot assays to examine the expression of CBS and CSE ( Fig. 1a–c , Supplementary Information ). The results showed that CBS and CSE were expressed in the human fallopian tube. Next, we investigated the cellular localization of the two different enzymes in the human oviduct by immunofluorescence staining or diaminobenzidine (DAB) staining in human oviduct slices. Confocal microscopy of the stained tissues showed that CBS and CSE were distributed in the human fallopian tube epithelium ( Fig. 1d–f ). The results from DAB staining further confirmed these findings ( Fig. 1g ). To determine whether the human oviduct generates detectable amounts of H 2 S, we performed a methylene blue assay to measure the H 2 S level in oviduct homogenates. The results showed that the biosynthesis of H 2 S was significantly increased after incubation of tissue homogenates with L -Cys, the CBS/CSE substrate ( Fig. 1h ). D , L -propargylglycine (PAG), an inhibitor of CSE, and amino-oxyacetic acid (AOAA), an inhibitor of CBS, significantly and effectively blocked H 2 S production. Conversely, S -adenosyl- L -methionine (SAM), a CBS activator, largely enhanced the production of H 2 S. These findings show that the human oviduct is capable of synthesizing H 2 S and that, under normal conditions, H 2 S is endogenously produced in the human oviduct. 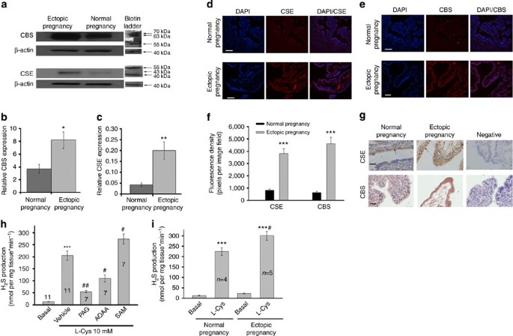Figure 1: A H2S generation pathway exists in the human fallopian tube. All data are mean±s.e.m. (a) Representative western blot analysis for CBS and CSE. (b,c) Comparison of the relative CBS or CSE amount expressed in human fallopian tube between the ectopic (n=5) and normal pregnancy groups (n=4). *P<0.05; **P<0.01 versus normal pregnancy group (unpairedt-test). (d,e) Typical immunofluorescence images showing the cellular distribution of CSE (d, red) or CBS (e, red) in a human fallopian tube. Scale bar, 20 μm. Semi-quantitative analysis of immunofluorescence staining shown as the fluorescent pixels per image field. (f) The summaries of the fluorescence densities of CSE and CBS in the fallopian tube epithelium of normal pregnant women (n=16 image fields of eight slices from four samples) and ectopic pregnant women (n=20 image fields of ten slices from five samples). ***P<0.001 versus normal pregnancy ( pairedt-test). (g) DAB staining of CBS and CSE in oviduct slices from human. Scale bar, 20 μm. The black arrows indicate the positive staining of the epithelium. (h) Human oviduct homogenate produced H2S. Incubation of oviduct homogenate with 10 mML-Cys caused a significant increase in H2S production compared with basal values (n=11 excised human fallopian tube samples). ***P<0.001 versus basal (pairedt-test). PAG (1 mM) or AOAA (1 mM) significantly inhibited theL-Cys-induced increase in H2S production, whereas SAM enhanced the production of H2S (n=7–11 excised human fallopian tube samples).#P<0.05;##P<0.01 versus vehicle (unpairedt-test). The expression of H2S-synthesizing enzymes CBS and CSE was upregulated in the fallopian tube with an ectopic pregnancy compared with the normal pregnancy (a–g). (i) The production of H2S was increased in the fallopian tube with an ectopic pregnancy compared with the normal pregnancy.n=4–5 excised human fallopian tube samples; ***P<0.001 versus basal conditions (pairedt-test);#P<0.05 versus normal pregnancy (unpairedt-test). Figure 1: A H 2 S generation pathway exists in the human fallopian tube. All data are mean±s.e.m. ( a ) Representative western blot analysis for CBS and CSE. ( b , c ) Comparison of the relative CBS or CSE amount expressed in human fallopian tube between the ectopic ( n =5) and normal pregnancy groups ( n =4). * P <0.05; ** P <0.01 versus normal pregnancy group (unpaired t -test). ( d , e ) Typical immunofluorescence images showing the cellular distribution of CSE ( d , red) or CBS ( e , red) in a human fallopian tube. Scale bar, 20 μm. Semi-quantitative analysis of immunofluorescence staining shown as the fluorescent pixels per image field. ( f ) The summaries of the fluorescence densities of CSE and CBS in the fallopian tube epithelium of normal pregnant women ( n =16 image fields of eight slices from four samples) and ectopic pregnant women ( n =20 image fields of ten slices from five samples). *** P <0.001 versus normal pregnancy ( paired t -test). ( g ) DAB staining of CBS and CSE in oviduct slices from human. Scale bar, 20 μm. The black arrows indicate the positive staining of the epithelium. ( h ) Human oviduct homogenate produced H 2 S. Incubation of oviduct homogenate with 10 mM L -Cys caused a significant increase in H 2 S production compared with basal values ( n =11 excised human fallopian tube samples). *** P <0.001 versus basal (paired t -test). PAG (1 mM) or AOAA (1 mM) significantly inhibited the L -Cys-induced increase in H 2 S production, whereas SAM enhanced the production of H 2 S ( n =7–11 excised human fallopian tube samples). # P <0.05; ## P <0.01 versus vehicle (unpaired t -test). The expression of H 2 S-synthesizing enzymes CBS and CSE was upregulated in the fallopian tube with an ectopic pregnancy compared with the normal pregnancy ( a – g ). ( i ) The production of H2S was increased in the fallopian tube with an ectopic pregnancy compared with the normal pregnancy. n =4–5 excised human fallopian tube samples; *** P <0.001 versus basal conditions (paired t -test); # P <0.05 versus normal pregnancy (unpaired t -test). Full size image H 2 S signalling is upregulated in oviductal pregnancy To investigate whether CBS or CSE/H 2 S activity is altered in oviductal pregnancy, we tested the expression of the H 2 S-producing enzymes, CBS and CSE, in a human fallopian tube with an ectopic pregnancy. Our results revealed that both enzymes were upregulated in the fallopian tube with an ectopic pregnancy compared with a normal pregnancy ( Fig. 1a–f ). Using the enzymatic H 2 S production assays, we further confirmed the upregulation of H 2 S production in ectopic pregnancy ( Fig. 1i ). H 2 S signalling regulates tubal contractility The oviduct plays an essential role during female reproduction by regulating the transport of gametes and embryos, and it provides a specific microenvironment for fertilization and the primary stages of embryonic development [16] . Our study yielded the following key findings: first, the human oviduct possesses both CBS and CSE proteins; second, homogenates of the human oviduct convert L -Cys (the substrate) to H 2 S; third, PAG and AOAA inhibit L -Cys conversion; and, finally, both enzymes are localized in the epithelium of the human fallopian tube. On the basis of these findings, we performed a functional study using isolated fallopian tube strips. Under normal conditions, the smooth muscle strips of the fallopian tube exhibited a regular, sphincter-like pattern of contractile activity ( Fig. 2a ). Exogenous application of H 2 S donor sodium hydrosulphide (NaHS, 10 −3 M) caused an immediate but sustained relaxation in 57 of 57 strips from 26 women. L -Cys (10 mM), a substrate of CBS/CSE, also inhibited contractile activity in 12 of 15 strips from seven women ( Fig. 2 ). In some experiments, a dose-related effect response of NaHS or L -Cys was observed ( Fig. 3 , n =5–7 strips from five women). We next investigated the effects of inhibitors of H 2 S synthesis on the spontaneous contraction of human fallopian tube. PAG (1 mM) increased the basal tone of spontaneous motility ( Fig. 4a,d ). AOAA (1 mM) caused an increase in the phasic contraction ( Fig. 4b,e,f ), whereas a CBS activator, SAM, reduced the spontaneous motility of the human fallopian tube ( Fig. 4c,g,h ). These responses were observed in 15 of 19 strips from seven women. Our data suggest that enzymatic production of H 2 S regulates fallopian tube motility. Taken together, these results demonstrated that endogenous H 2 S plays a relaxant role in the regulation of muscular contractions in the human fallopian tube. Thus, we provide the first evidence of the presence H 2 S in the human oviduct, as well as demonstrating a physiological role for H 2 S in regulating tubal contractility. 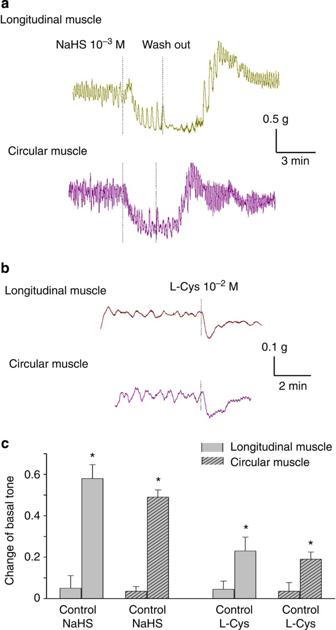Figure 2: Effect of NaHS orL-Cys on the contractile activity of human fallopian tube strips. (a) Representative trace of NaHS orL-Cys-induced inhibition on contractile activity of human fallopian tube strips. NaHS caused a decrease in the basal tone of human fallopian tube spontaneous contractions, and this response could be completely washed out. (b)L-Cys also decreased the basal tone. (c) Summary of the changes in basal tone induced by NaHS (n=57 tissue strips from 26 women) orL-Cys (n=12 tissue strips from seven women). All data are mean±s.e.m., *P<0.05 versus control (pairedt-test). Figure 2: Effect of NaHS or L -Cys on the contractile activity of human fallopian tube strips. ( a ) Representative trace of NaHS or L -Cys-induced inhibition on contractile activity of human fallopian tube strips. NaHS caused a decrease in the basal tone of human fallopian tube spontaneous contractions, and this response could be completely washed out. ( b ) L -Cys also decreased the basal tone. ( c ) Summary of the changes in basal tone induced by NaHS ( n =57 tissue strips from 26 women) or L -Cys ( n =12 tissue strips from seven women). All data are mean±s.e.m., * P <0.05 versus control (paired t -test). 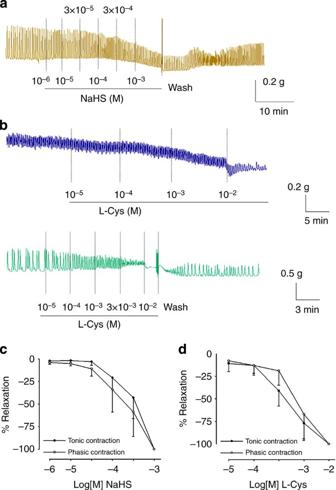Figure 3: Concentration-dependent effects of NaHS orL-Cys on contractile activity of human fallopian tube strips. (a,b) Representative trace of the NaHS orL-Cys-induced dose-dependent inhibition of contractile activity of human fallopian tube strips. NaHS (1 μM–1 mM) orL-Cys (10 μM–10 mM) caused a dose-dependent relaxation. (c,d) Summary of dose-dependent effect induced by NaHS (c,n=7 tissue strips of oviduct from five women) orL-Cys (D,n=5 tissue strips from five women). All data are mean±s.e.m. Full size image Figure 3: Concentration-dependent effects of NaHS or L -Cys on contractile activity of human fallopian tube strips. ( a , b ) Representative trace of the NaHS or L -Cys-induced dose-dependent inhibition of contractile activity of human fallopian tube strips. NaHS (1 μM–1 mM) or L -Cys (10 μM–10 mM) caused a dose-dependent relaxation. ( c , d ) Summary of dose-dependent effect induced by NaHS ( c , n =7 tissue strips of oviduct from five women) or L -Cys (D, n =5 tissue strips from five women). All data are mean±s.e.m. 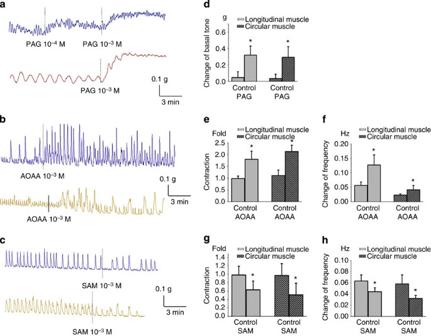Figure 4: Effects of the inhibitors and activator of H2S-synthesizing enzymes on contractile activity of human fallopian tube strips. (a) Representative traces of effect of PAG, an inhibitor of CSE, (b) AOAA, an inhibitor of CBS and (c) SAM, an activator of CBS, on the contractile activity of the human fallopian tube strips. (d–h) Summary of the effects of PAG, AOAA and SAM on spontaneous contractile activity of the human fallopian tube strips (n=15 tissue strips from seven women for each group). All data are mean±s.e.m., *P<0.05 versus control (pairedt-test). Full size image Figure 4: Effects of the inhibitors and activator of H 2 S-synthesizing enzymes on contractile activity of human fallopian tube strips. ( a ) Representative traces of effect of PAG, an inhibitor of CSE, ( b ) AOAA, an inhibitor of CBS and ( c ) SAM, an activator of CBS, on the contractile activity of the human fallopian tube strips. ( d – h ) Summary of the effects of PAG, AOAA and SAM on spontaneous contractile activity of the human fallopian tube strips ( n =15 tissue strips from seven women for each group). All data are mean±s.e.m., * P <0.05 versus control (paired t -test). Full size image Dysregulation of H 2 S metabolism impairs embryo transport As noted above, H 2 S can be produced in the human fallopian tube, which acts as a regulator of fallopian tube motility. In rodents, embryos are rapidly transported through the oviduct ampulla, but slow down once they reach the ampulla-isthmus junction, and they reside at the isthmus for ~3 days. Embryos transport from this region into the uterus aided by a wave of regulated contraction and relaxation of the oviduct muscularis. Thus, muscular activity of the isthmus is the main contributor to oviductal embryo transport. Hypothesizing that H 2 S signalling might be involved in tubal egg transport, we tested its effect on oviductal embryo transport in pregnant mice. As expected, after administration of NaHS or GYY4137 (H 2 S donor), AOAA (a specific CBS inhibitor ) and SAM (a CBS activator), 7 of 27 mice did not yield any embryos when their uterine lumens were flushed at midmorning of day 4 of pregnancy. However, embryos at the morula stage were recovered from the oviducts of these mice ( Fig. 5a,b ). The development of embryos from treatment mice was asynchronous compared with the control group. As expected, more than 93% of the control embryos recovered from the uterus at this time were blastocysts. However, less than 20% of the treatment embryos (either NaHS or GYY4137) were at the blastocyst stage, and a larger number of embryos were at the morula stage ( Fig. 5c,d ). In the other treatment group, half of the embryos were at the blastocyst stage. These findings provide evidence that if H 2 S signalling is abnormal or dysregulated, oviductal embryo transport and early embryo development are delayed, thereby preventing timely implantation in the uterus. Unexpectedly, compared with control subjects, PAG, an inhibitor of CSE, did not affect the oviductal embryo transport, although the delay of early embryo development was still observed. Previous studies have demonstrated that CBS (−/−) females are infertile [17] , [18] ; therefore, in our study, we used CBS(+/−) mice to investigate the role of H 2 S signalling in early embryo transport. The results showed that the embryos retained in the oviduct were observed in the midmorning of day 4 of pregnancy in the CBS (+/−) females mated with wild-type males compared with wild-type females. Furthermore, the development of embryos was also asynchronous ( Fig. 5e–g ). The accumulating data suggested that embryo-maternal communication exists in the preimplantation period [19] . To exclude the role of CBS (+/−) embryos on the oviduct motility, we used wild-type females mated with CBS (+/−) males. Our results showed that no embryo was retained in the oviduct, although the development of embryos was also asynchronous, demonstrating that this effect on oviductal embryo transport is independent of embryonic CBS. These results provide genetic evidence that oviductal CBS directs the timely oviductal transport of embryos. Collectively, these observations support the idea that aberrant H 2 S signalling, which arises from either silencing or amplification, impedes the coordinated oviductal smooth muscle contraction and relaxation that are critical to normal embryo transport during early pregnancy. We speculated that balancing the H 2 S signalling would help to normalize oviductal embryo transport in either AOAA-treated mice or CBS(+/−) mice. Indeed, administration of GYY4137, a slow-releasing H 2 S donor, or NaHS rescues the impaired embryo transport or the asynchronous development in these mice ( Fig. 6 ). 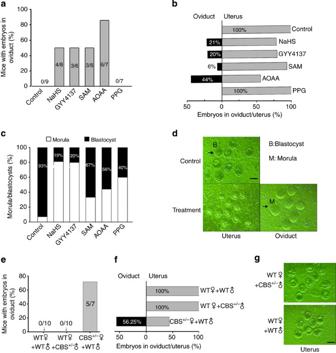Figure 5: Pharmacological or genetic intervention for CBS prevented oviductal embryo transport and early embryo development. (a) Number of mice with oviductal retention of embryos/total number of BALB/c mice examined. (b) Percentage of embryos recovered from oviducts or uteri. (c) Differential distribution of morulae and blastocysts for different treatments. (d) Morphology of embryos recovered from oviducts or uteri. Both morulae and blastocysts were recovered from the oviducts or uteri of mice treated with drugs or control (non-drug-treated) mice on day 4 midmornings. Scale bar, 100 μm. (e) Number of mice with oviductal retention of embryos/total number of CBS+/−mice or wild-type mice examined. (f) Percentage of embryos recovered from oviducts or uteri of CBS+/−mice or wild-type mice. (g) Morphology of embryos recovered from oviducts or uteri of CBS+/−mice or wild-type mice. Scale bar, 100 μm. Figure 5: Pharmacological or genetic intervention for CBS prevented oviductal embryo transport and early embryo development. ( a ) Number of mice with oviductal retention of embryos/total number of BALB/c mice examined. ( b ) Percentage of embryos recovered from oviducts or uteri. ( c ) Differential distribution of morulae and blastocysts for different treatments. ( d ) Morphology of embryos recovered from oviducts or uteri. Both morulae and blastocysts were recovered from the oviducts or uteri of mice treated with drugs or control (non-drug-treated) mice on day 4 midmornings. Scale bar, 100 μm. ( e ) Number of mice with oviductal retention of embryos/total number of CBS +/− mice or wild-type mice examined. ( f ) Percentage of embryos recovered from oviducts or uteri of CBS +/− mice or wild-type mice. ( g ) Morphology of embryos recovered from oviducts or uteri of CBS +/− mice or wild-type mice. Scale bar, 100 μm. 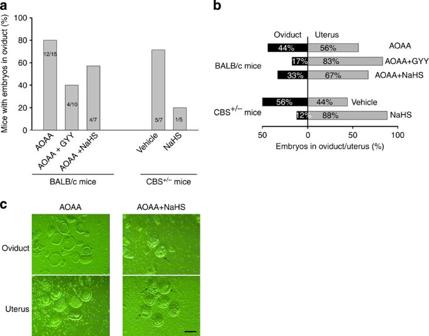Figure 6: Impaired oviductal embryo transport in BALB/c mice treated with AOAA or CBS+/−mice was rescued by the H2S donors NaHS or GYY4137. (a) Number of mice with oviductal retention of embryos/total number of mice examined. (b) Percentage of embryos recovered from oviducts or uteri. (c) Differential distribution of morulae and blastocysts for different treatments. GYY4137: 10 mg kg−1; NaHS: 0.5 mg kg−1. Black arrow indicates blastocyst. Scale bar, 100 μm. Full size image Figure 6: Impaired oviductal embryo transport in BALB/c mice treated with AOAA or CBS +/− mice was rescued by the H 2 S donors NaHS or GYY4137. ( a ) Number of mice with oviductal retention of embryos/total number of mice examined. ( b ) Percentage of embryos recovered from oviducts or uteri. ( c ) Differential distribution of morulae and blastocysts for different treatments. GYY4137: 10 mg kg −1 ; NaHS: 0.5 mg kg −1 . Black arrow indicates blastocyst. Scale bar, 100 μm. Full size image This is the first report to provide evidence that H 2 S-synthesizing enzymes CBS and CSE are distributed in the human fallopian tube and that production of H 2 S regulates contraction in excised human fallopian tube samples and is required for transport of the embryo through the fallopian tube in mice. Importantly, an aberration in H 2 S signalling, including silenced or enhanced activity induced by pharmacologic or genetic methods, causes embryo retention and developmental delay in the mouse oviduct. Our study provides a new regulatory mechanism for oviductal transport of embryos and early embryonic development. Expression of CSE or CBS is tissue specific. CSE is expressed predominantly in peripheral vascular tissues and the heart, whereas CBS is highly expressed in the central and peripheral nervous systems [20] , [21] . In the present study, we demonstrated that both CSE and CBS were expressed primarily in the human oviduct epithelium. H 2 S has been shown to cause relaxation of arterial blood vessels [2] , [21] , [22] , small bronchial rings [23] , [24] , [25] , human corpus cavernosum [7] , rat vas deferens [11] , and gastrointestinal and urogenital smooth muscle [26] . The human fallopian tube is capable of synthesizing H 2 S. In our in vitro experiments, the production of H 2 S also relaxed the spontaneous contraction of the human oviduct, which suggests that an endogenous H 2 S relaxation system functionally exists in the fallopian tube. The oviduct’s normal function is to pick up the ovulated oocytes, convey them to the ampulla for fertilization, and then transport the preimplantation embryos to the uterus at a precisely regulated rate for implantation [27] , [28] . Factors that interfere with oocyte pick up, fertilization or preimplantation embryo transport can impede the establishment of a normal pregnancy. The incidence of ectopic pregnancy has significantly increased in recent decades [29] . Ectopic pregnancy results from a delay in the passage of the fertilized ovum through the fallopian tube. This delay can result from anatomical abnormalities of the tubes or from tubal dysfunction, including altered contractility or abnormal ciliary activity. Approximately 95% of ectopic pregnancies occur in the tubes, and most are located in the distal parts, particularly the ampulla. Embryo retention in the fallopian tube as a result of dysfunctional muscular contraction is one cause of ectopic pregnancy [30] . As mentioned above, H 2 S is a mediator of oviductal contractility. Dysregulation of H 2 S homeostasis has also been implicated in numerous pathological conditions and diseases. In our present study, we found that H 2 S signalling is upregulated in the human fallopian tube with an ectopic pregnancy, which suggests that dysregulation of H 2 S metabolism is involved. The oviductal smooth muscle contraction and relaxation are coordinated, which is essential for oviductal embryo transport during early pregnancy. An aberration in H 2 S signalling by silenced or enhanced activity induced by pharmacologic or genetic methods retards embryo transport. Some studies have indicated that the physiological role of CBS-derived H 2 S differs from that of CSE-derived H 2 S. In the liver, CBS-derived H 2 S regulates lipopolysaccharide (LPS)-induced apoptosis of hepatic cells [31] , whereas CSE-derived H 2 S has been associated with the pathogenesis of hypertension [21] . CSE-knockout mice are fertile and give birth normally [21] . Conversely, CBS is essential for female reproductive function. Female offspring of CBS-knockout mice have reduced fertility, whereas male offspring are fertile [17] , [18] . In our in vitro experiment, the isolated strips of the human fallopian tube exhibited both phasic and tonic contractile activity. Intriguingly, CSE-derived H 2 S regulates the tone of spontaneous motility, whereas CBS-derived H 2 S mediates the phasic contraction. Furthermore, we observed in our in vivo study that CBS-derived H 2 S, but not CSE-derived H 2 S, was involved in embryo transport, which was consistent with previous research indicating that CBS is essential for female reproductive function [17] , [18] , [21] . Both CBS and CSE are localized in the cytosol [32] . However, the subcellular compartmentalization of H 2 S produced by these enzymes may be different. Compartmentalization of sulphur stores may facilitate differential H 2 S release for specialized purposes. In addition, the expression of CBS in the human fallopian tube is higher than that of CSE ( Fig. 1 ). Therefore, we speculate that the differential effects of CBS-derived H 2 S and CSE-derived H 2 S on oviductal contractility or embryo transport may be caused by different subcellular localizations or different concentrations of these two enzyme-derived H 2 S. Furthermore, we found that H 2 S signalling is involved in preimplantation embryo development. Both CBS-derived H 2 S and CSE-derived H 2 S delay early embryo development, although they have different roles in oviductal function. Embryo-maternal communication exists in the preimplantation period [19] . Interestingly, embryonic CBS-derived H 2 S contributes primarily to normal embryo development but not to the function of the maternal oviduct. Our work demonstrates that under normal physiological conditions, H 2 S signalling is crucial to oviductal transport and early embryo development. Conversely, an aberration in H 2 S signalling, whether silenced or enhanced, derails these processes. Western blots Human fallopian tubes were obtained via salpingectomies for ectopic pregnancy, and hysterectomy or postpartum sterilization samples collected from women aged 23–48 years who had not undergone exogenous hormonal treatment for at least 3 months before surgery. All donors were considered fertile. Written informed consent was obtained from each patient, and approval was granted by the Medical Ethics Committees of Shandong University (number MECSDUMS 2010032). Human oviduct tissue was homogenized in modified RIPA buffer (50 mM Tris-HCl pH 7.4, 1% Triton X-100, 0.25% Na-deoxycholate, 150 mM NaCl, 1 mM EDTA, 1 mmol l −1 PMSF, 10 mg ml −1 aprotinin, 20 μmol l −1 leupeptin and 50 mM NaF). After centrifugation of homogenates at 12,000 r.p.m. for 20 min at 4 °C, to the supernatant was added the same amount of sample buffer boiled 10 min at 100 °C. Ten to thirty μg of denatured proteins were separated on 10% SDS polyacrylamide gels and transferred to a PVDF membrane. Membranes were blocked in a blocking buffer (containing 5% non-fat dry milk and Tween-Tris-buffered saline) for 1 h at room temperature, then washed in Tween-Tris-buffered saline (0.1% Tween 20, 50 mM Tris and 150 mM NaCl), followed by overnight incubation at 4 °C with a rabbit polyclonal CBS antibody (Santa Cruz Biotechnology, Santa Cruz, CA, 1:500 dilution) or a rabbit polyclonal CSE antibody (Abcam, Cambridge, UK, 1:500 dilution). Membranes were washed in Tween-Tris-buffered saline and incubated with an anti-horseradish-peroxidase-conjugated secondary antibody (1:4,000). The membranes were washed again and exposed to ECL. The blot films were scanned, and the band densities were calculated using the Quantity One analysis software (Bio-Rad). The values of blot densities were normalized to the levels of respective β-actin blots. Immunofluorescence Paraffin sections were roasted 90 min at 65 °C, dewaxed in xylene twice for 10 min and then rehydrated in 100, 100, 95, 95, 90 and 80% of ethanol and running tap water for 5 min each, in order. Tissue sections underwent antigen retrieval in a solution consisting of 0.01 M citrate and 0.01 M sodium citrate before they were blocked in PBS containing 10% goat serum for 1 h at room temperature. The sections were incubated with a polyclonal CBS antibody (Santa Cruz Biotechnology, Santa Cruz, CA, 1:100 dilution) or polyclonal CSE antibody (Abcam, Cambridge, UK, 1:100 dilution) overnight at 4 °C After being washed in PBS, the sections were incubated with Alexa Fluor 568 goat anti-rabbit IgG (H+L) (1: 600; Invitrogen Carlsbad, CA, USA) for 1 h at room temperature. The sections were washed again and incubated in DAPI (1:1,000) for 10 min at room temperature. In negative controls, the sections were incubated with PBS instead of the primary antibody. We repeated the immunohistochemistry of each protein in eight tissue slices of four samples. The fluorescence intensity for a specific protein stain was set below the threshold for the negative control. DAB staining The cross-section of human fallopian tube samples was cut (4 μm) and used for CSE and CBS immunohistochemistry. Sections were stained using a two-step method. Activity of endogenous peroxidase was blocked with 3% hydrogen peroxide. After three rinses in PBS, 10% normal rabbit serum was applied for 15 min, and then the sections were incubated with the polyclonal CBS antibody (Santa Cruz Biotechnology, Santa Cruz, CA, 1:100 dilution) or polyclonal CSE antibody (Abcam, Cambridge, UK, 1:100 dilution) overnight in a humid chamber at 4 °C. After the sections were washed, they were incubated with polymer peroxidase anti-rabbit serum for 30 min at room temperature. After several rinses, peroxidase was revealed by using a 3,3-diaminobenzidine tetrahydrochloride substrate kit (ZSGB-BIO). Preparation of muscle strips Segments of the human oviduct were immediately removed and placed in a glass beaker containing 4 °C Krebs solution. The transverse and longitudinal muscle strips of the human oviducts were prepared. The isolated smooth muscle strips were placed in isolated organ baths filled with Krebs solution, which contained 95% O 2 and 5% CO 2 , incubated and connected with tension transducers. The Krebs solution contained the following: 5.9 mM KCl, 1.2 mM NaH 2 PO 4 , 1.2 mM MgCl 2 , 120.6 mM NaCl, 15.4 mM NaHCO 3 , 11.5 mM glucose and 2.5 mM CaCl 2 . The strips were stretched and reached a resting tension of 1 g. Until the tension was recorded, the strips needed to equilibrate for 30 min, as necessary, and the bathing solution was periodically changed. Subsequently, NaHS, L -Cys, PAG, AOAA and SAM were added, and the respective contraction curve was recorded. Whenever the reagents were replaced, the tissues were washed three times. The release of H 2 S The tissue H 2 S production rate was measured as described previously [33] . In brief, human fallopian tube samples were homogenized in 50 mM ice-cold potassium phosphate buffer pH 6.8. The reaction mixture contained (mM): 10% (w/v) tissue homogenate (0.5 ml), 100 potassium phosphate buffer pH 7.4 (0.5 ml), 2 pyridoxal 5′-phosphate (0.1 ml) and 10 L -cysteine (0.1 ml). Cryovial test tubes (2 ml) were used as the centre wells, and each well contained 0.5 ml 1% zinc acetate as the trapping solution. The reaction was performed in a 25-ml flask containing the reaction mixture and the centre well. Before being sealed, the flask was flushed with N 2 . The reaction was initiated by transferring the flasks from ice to a 37 °C shaking water bath. After incubation at 37 °C for 90 min, trichloroacetic acid (50%, 0.5 ml) was added to the reaction mixture to stop the reaction and incubated at 37 °C for an additional 60 min. The contents of the centre wells were then transferred to test tubes, each containing 3.5 ml of ultra-pure water. Subsequently, 0.5 ml of 20 mM N,N -dimethyl-p-phenylenediamine sulphate in 7.2 M HCl was added, immediately followed by the addition of 0.4 ml 30 mM FeCl 3 . After 20 min of incubation at room temperature, the optical absorbance of the resulting solutions was measured at 670 nm. The H 2 S concentration was calculated against the calibration curve of the standard H 2 S solutions. Embryo transport BALB/c mice were purchased from the Animal Center, Shandong University, China. Wild-type (WT) and CBS +/− mice on a C57BL/6J background were obtained from the Jackson Laboratory (Bar Harbor, ME). All the animal experiments were approved by the Medical Ethics Committee of Shandong University (number ECAESDUSM 2012029). Female mice (6–8 weeks of age) were mated randomly, and vaginal plug-positive mice were used in the experiment. Pregnant mice were divided into eight groups and given drugs as follows: saline ( n =9), NaHS (5 mg kg −1 , Sigma, n =8), GYY4137 (50 mg kg −1 , Cayman Chemical, n =6), SAM (50 mg kg −1 , Sigma, n =6), AOAA (50 mg kg −1 , Sigma, n =22), PAG (100 mg kg −1 , Sigma, n =7), AOAA (50 mg kg −1 kg)+ GYY4137 (10 mg kg −1 ) ( n =10) and AOAA (50 mg kg −1 )+ NaHS (0.5 mg kg −1 ) ( n =7). Each pregnant mouse received four intraperitoneal injections at 0, 24, 48 and 72 h after the discovery of the vaginal plug. The mice were killed via cervical dislocation at 74 h after the discovery of the vaginal plug, and the oviducts and uterus were placed in 1.0 ml saline, respectively. The embryos were flushed with 0.4 ml saline from the oviducts or uteri and counted. Statistical analysis Statistical analyses were performed with Sigmaplot software (SPSS). Data are expressed as the mean±s.e.m. and were examined with Student’s unpaired or paired t -tests where appropriate. A P -value of <0.05 was considered significant. How to cite this article: Ning, N. et al. Dysregulation of hydrogen sulphide metabolism impairs oviductal transport of embryos. Nat. Commun. 5:4107 doi: 10.1038/ncomms5107 (2014).